Genome-wide association study ofArabidopsis thalianaleaf microbial community Identifying the factors that influence the outcome of host–microbial interactions is critical to protecting biodiversity, minimizing agricultural losses and improving human health. A few genes that determine symbiosis or resistance to infectious disease have been identified in model species, but a comprehensive examination of how a host genotype influences the structure of its microbial community is lacking. Here we report the results of a field experiment with the model plant Arabidopsis thaliana to identify the fungi and bacteria that colonize its leaves and the host loci that influence the microbe numbers. The composition of this community differs among accessions of A. thaliana . Genome-wide association studies (GWAS) suggest that plant loci responsible for defense and cell wall integrity affect variation in this community. Furthermore, species richness in the bacterial community is shaped by host genetic variation, notably at loci that also influence the reproduction of viruses, trichome branching and morphogenesis. Plants, the main driver of primary productivity in terrestrial ecosystems, provide habitat to countless bacteria, yeasts, filamentous fungi, protists, oomycetes and nematodes. Recent studies have investigated the role of the environment and host-genetics in affecting the bacteria that live in both the rhizosphere [1] , [2] , [3] , [4] , [5] and phyllosphere [6] , [7] , [8] , [9] . The discovery that these communities are shaped, at least in part, by host genetic variation motivates the search for the host genes involved [2] , [3] , [4] , [6] , [9] . The plant genetic model, A. thaliana , is ideal for investigating the molecular bases of traits of ecological and agricultural interest, including resistance to fungal and bacterial species, and has been used successfully to identify loci that recognize individual isolates of model pathogens [10] , [11] . Here we investigate which microbial species colonize the leaves of A. thaliana and whether host-genetic factors play a discernible role. 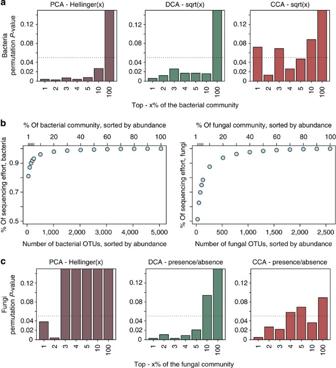Figure 1: Genetic variation withinA. thalianashapes the composition of the best-sequenced members of the microbial community. (a) Using eigenvector techniques, inbred replicates ofA. thalianacluster together only when analysing the most heavily sequenced bacteria. Nevertheless, the vast majority of the sequencing effort characterizes a small number (and %) of taxa in each community. (b) Taken together, this implies that vagrant species and other poorly characterized/sequenced taxa (and occasionally, sequencing artefacts) obscure evidence that hosts shape their microbial communities. (c) Host-genetic variation withinA. thalianaalso affects the ability of fungi to colonize and proliferate on its leaves. AllPvalues take into account technical confounders. For this purpose, we grew a worldwide diversity panel of 196 accessions [10] ( Supplementary Table 1 ), in replicate, in a field site where the species occurs. To be consistent with the predominantly winter-annual life history of A. thaliana , we conducted our experiment from autumn to spring, and at the end of the experiment took a ‘snapshot’ of the microbial community by flash-freezing samples in the field. Here, in addition to characterizing the bacteria and fungi that live in the leaves of A. thaliana , we identify the host genes that contribute to the structure of its microbial community. The leaf microbial community of A. thaliana Leaves were washed and vortexed to remove loosely associated microbes before extracting DNA from each leaf rosette. To characterize the bacterial community in each sample, variable regions 5 (V5), 6 and 7 of bacterial 16S ribosomal DNA (rDNA) genes were PCR-amplified using the primer pair 799F and 1193R. In addition, the first internal transcribed spacer (ITS1) within eukaryotic rDNA was amplified using the fungal-specific primer ITS1-F with ITS2. All amplicons were sequenced, in multiplex, using a 454 FLX system (Titanium chemistry). After basic quality control (Methods), ~3,186±2,202 (mean±s.d.) bacterial reads (1,768,402 total reads) and ~526±248 fungal reads (297,871 reads) were obtained from each sample. DNA sequences sharing ≥97% pairwise similarity were clustered to identify species-level operational taxonomic units (OTUs). Across accessions, we found 5,057 non-singleton bacterial OTUs, with the majority belonging to families in the Proteobacteria, Bacteroidetes and Actinobacteria ( Supplementary Fig. 1a–d ). In particular, Sphingomonas (α-proteobacteria), Flavobacterium (Bacteroidetes), Rhizobium (α-proteobacteria) and Pseudomonas (γ-proteobacteria)—all of which are known to occur in the phyllosphere of A. thaliana throughout much of the species range [12] , [13] —were common genera. A total of 2,582 non-singleton fungal OTUs were also observed, mostly representing families from the ascomycete classes Dothideomycetes and Sordariomycetes, and the basidiomycete class Tremellomycetes ( Supplementary Fig. 1e–h ). Genera known to contain plant pathogens included Epicoccum , Alternaria , Mycosphaerella , Fusarium and Plectosphaerella . The most heavily sequenced (that is, most ‘abundant’) fungal OTUs share taxonomic affinity with the genus Tetracladium , which, although originally assumed to be restricted to aquatic environments, are frequently found on plants [14] . After correcting for differences in sequencing among samples and adjusting for technical confounders, strong and significant species associations (Kendall’s Test of Concordance [15] , P =0.001, 1,000 permutations) were observed within both the bacterial and fungal communities ( Supplementary Figs 2 and 3 ), suggesting that members of the microbial community interact or that portions of the microbial community respond to the same host factors. To take into account these correlations, we summarized each community using eigenvector techniques (Methods), including principal component analysis (PCA) and canonical correspondence analysis (CCA). The leaf microbial community is shaped by host genetics We found that genetic variation within A. thaliana clearly shapes the leaf bacterial community, but only when we focused on the most heavily sequenced OTUs. As an example, PCA of the bacterial community distinguishes accessions of A. thaliana according to host-genotype, with inbred replicates of the same accession significantly clustered together ( Fig. 1a ; Methods) when analysing, at most, the top 50% of the community ( H 2 ~40%; P =0.044, 1,000 permutations; for the top 1%, H 2 ~42%; P =0.004). However, these 2,528 bacterial OTUs correspond to >99% of the sequencing reads, which suggests that rare species or sequencing artefacts [16] , [17] may obscure evidence that hosts structure their microbial communities ( Fig. 1b ). Figure 1: Genetic variation within A. thaliana shapes the composition of the best-sequenced members of the microbial community. ( a ) Using eigenvector techniques, inbred replicates of A. thaliana cluster together only when analysing the most heavily sequenced bacteria. Nevertheless, the vast majority of the sequencing effort characterizes a small number (and %) of taxa in each community. ( b ) Taken together, this implies that vagrant species and other poorly characterized/sequenced taxa (and occasionally, sequencing artefacts) obscure evidence that hosts shape their microbial communities. ( c ) Host-genetic variation within A. thaliana also affects the ability of fungi to colonize and proliferate on its leaves. All P values take into account technical confounders. Full size image Species of bacteria tend to be more prevalent (that is, common) across host samples than species of fungi, leading to higher estimates of turnover (β-diversity) in the fungal than bacterial community ( Supplementary Fig. 4 ). It is unclear whether fungi disperse poorly compared with bacteria, or whether other factors (for example, host selection and/or interspecific competition) differentially shape these two communities. Nevertheless, both presence/absence and abundance data reveal clear evidence that host-genetic variation shapes the communities of fungi associated with the leaves of A. thaliana , but for only the most heavily sequenced taxa ( Fig. 1c ). We looked for further evidence that hosts shape their microbial communities by using genome-wide single-nucleotide polymorphism (SNP) data [18] to estimate the relatedness among accessions, before asking whether more closely related individuals harbour more similar communities. 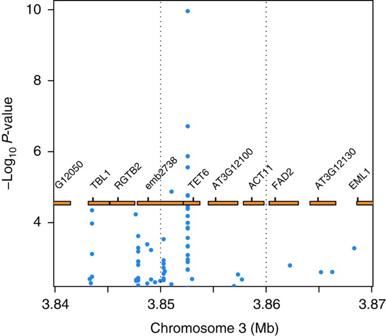Figure 2: The most frequently observed genomic region in the results from GWAS of the 100 most heavily sequenced bacterial OTUs. The points illustrate the minimumPvalue, per 10-kb region, from these separate analyses (that is, separate GWAS of individual OTUs), and this region is shared in the extreme tail for 9 out of these 100 OTUs (100,000 permutations;P=1 × 10−5). Notablea prioricandidate genes includeFAD2andTBL1; as mentioned in the main text, theTBLgene family is involved in secondary cell wall synthesis and cellulose deposition. The association peaks, however, onTETRASPANIN 6(TET6), a gene involved in metal ion transport. This approach is likely to underestimate the heritability of traits influenced by non-additive effects, genetic heterogeneity [19] , or by rare causal SNPs in incomplete linkage disequilibrium (LD) with genotyped SNPs [4] , [20] ; nevertheless, heritable eigenvectors were found in both communities, regardless of the ordination technique used (Methods; Supplementary Table 2 ). For example, SNPs explain 9% of the variance for PC1 ( P =0.003) and 8% of the variance for PC2 ( P =0.015) from PCA of the fungal community, as well as 11% of the variance for PC2 of the bacterial community ( P =0.001). The genes associated with the leaf microbial community Having established that microbial communities are shaped by host genotypes, we turned to GWAS [21] , [22] , [23] to map any major genetic variants underlying variation in these eigenvectors and, separately, the presence/absence and abundance of the most heavily sequenced ( n =100) taxa in each kingdom. In addition, to explore the processes shaping each microbial community, we used a false discovery rate (FDR) [24] of 10% to identify enriched gene ontology (GO) categories (Methods) [25] . We found that bacterial and fungal communities are shaped by similar biological processes, albeit by different underlying genes. In the analysis of individual OTUs, a few genomic regions stand out as being generally important ( Fig. 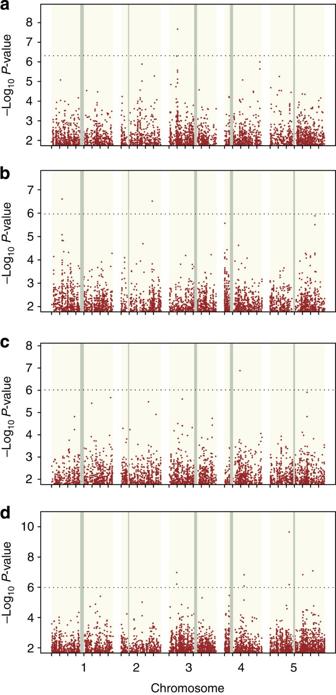Figure 3: Genes implicated in the community composition of the leaves. The ABC transporter C family members 7 and 8 (multidrug resistance-associated proteins 7 and 8) are associated (Chr 3, ~4.21 Mb) with the abundance of an OTU assigned toMycosphaerella(a), while ABC transporter G family member 35 (pleiotropic drug resistance 7; Chr 1, ~5.23 Mb) and a pectinesterase (AT2G36710; Chr 2, ~15.392 Mb) are implicated in the abundance of an OTU assigned toSphingomonas(b). Other pectin-related enzymes include the pectate lyase (AT4G13210; Chr 4, ~7.67 Mb) associated with the abundance ofChryseobacterium(c) and the pectinesterase (AT5G26810; Chr 5 ~9.432 Mb) associated with the abundance ofXanthomonas(d). Notablea prioricandidate genes also includeTERPENE SYNTHASE 10(TPS10; Chr 2, ~10.297 Mb) identified in (a), the resistance gene (R-gene) pinpointed (Chr 5, ~18.287 Mb) in (c), and the oxidoreductase (Chr 4, ~9.708 Mb) illustrated in (d). To assess genome-wide significance, a permutation approach was used that takes into account population structure (Methods). 2 and Supplementary Table 3 ), and candidate genes significantly overrepresented across analyses (Methods) tend to be associated with OTUs in only one kingdom (but see Supplementary Table 4 ). In contrast, gene set enrichment analyses reveal that the most common biological process overrepresented across analyses is ‘defense response’, followed closely by kinase-related activities, for both the bacterial and fungal community ( Table 1 ). Figure 2: The most frequently observed genomic region in the results from GWAS of the 100 most heavily sequenced bacterial OTUs. The points illustrate the minimum P value, per 10-kb region, from these separate analyses (that is, separate GWAS of individual OTUs), and this region is shared in the extreme tail for 9 out of these 100 OTUs (100,000 permutations; P =1 × 10 −5 ). Notable a priori candidate genes include FAD2 and TBL1 ; as mentioned in the main text, the TBL gene family is involved in secondary cell wall synthesis and cellulose deposition. The association peaks, however, on TETRASPANIN 6 ( TET6 ), a gene involved in metal ion transport. Full size image Table 1 Biological categories most often enriched in GWAS of the 100 most abundant OTUs. Full size table The cell wall, comprising the polysaccharides cellulose (β-1,4-glucan), callose (β-1,3-glucan) and pectin (a heteropolysaccharide), is one of the first obstacles for any plant pathogen, and biological processes associated with the cell wall are significantly overrepresented across GWAS of individual bacterial species. Similarly, for the combined fungal community, the strongest GWAS peaks for PC1 and PC2 from PCA each fall within candidate genes implicated in cell wall integrity. For PC1, the top SNP lies within GLUCAN-SYNTHASE-LIKE 11 ( GSL11 ); a related locus ( GSL5 ) in A. thaliana seals wounds that arise during fungal infection using callose [26] . For PC2, the top SNP falls within a member of the TRICHOME BIREFRINGENCE-LIKE gene family ( TBL37 ), which is involved in secondary cell wall formation through the deposition of cellulose [27] . Plant microtubules, which form the cytoskeleton and are regularly moved to the site of contact with a microbe, act as either a defense mechanism or, after reorganization of the plant cell wall, enable compatible symbioses with diverse microbial species [28] . Still other pathogens depolymerize microtubules to facilitate infection; in the case of viruses, microtubules provide a means for intra and intercellular mobility. Several distinct microtubule-related categories are significantly enriched in the results from GWAS of the fungal community ( Supplementary Table 5 ). Although many of the strongest associations are implicated in the presence/absence or abundance of only one or a few OTUs, several of these are members of large gene families, some of which are likely to be functionally redundant. For example, ATP-binding cassette (ABC) transporters ferry metabolites around the cell and across the cell membrane, and mutations in ABC transporters lead to various human diseases (for example, cystic fibrosis [29] ) and plant resistance to a number of toxins and pathogens [30] . ABC transporters are found among the strongest associations from GWAS of both bacterial and fungal OTUs (for example, Fig. 3a,b and Supplementary Table 4 ). As another example, pectin in the cell wall is frequently degraded by pathogen-produced enzymes (that is, pectinases) [31] . Even so, we found several (non-allelic) host polymorphisms involved in the synthesis and esterification of pectin to be associated with various OTUs ( Fig. 3b–d ), which highlights the role of cell wall integrity in shaping the composition of the leaf microbial community. The results from all analyses have been deposited in the Dryad Digital Repository ( http://doi.org/10.5061/dryad.8sm01 ). Figure 3: Genes implicated in the community composition of the leaves. The ABC transporter C family members 7 and 8 (multidrug resistance-associated proteins 7 and 8) are associated (Chr 3, ~4.21 Mb) with the abundance of an OTU assigned to Mycosphaerella ( a ), while ABC transporter G family member 35 (pleiotropic drug resistance 7; Chr 1, ~5.23 Mb) and a pectinesterase (AT2G36710; Chr 2, ~15.392 Mb) are implicated in the abundance of an OTU assigned to Sphingomonas ( b ). Other pectin-related enzymes include the pectate lyase ( AT4G13210 ; Chr 4, ~7.67 Mb) associated with the abundance of Chryseobacterium ( c ) and the pectinesterase ( AT5G26810 ; Chr 5 ~9.432 Mb) associated with the abundance of Xanthomonas ( d ). Notable a priori candidate genes also include TERPENE SYNTHASE 10 ( TPS10 ; Chr 2, ~10.297 Mb) identified in ( a ), the resistance gene ( R -gene) pinpointed (Chr 5, ~18.287 Mb) in ( c ), and the oxidoreductase (Chr 4, ~9.708 Mb) illustrated in ( d ). To assess genome-wide significance, a permutation approach was used that takes into account population structure (Methods). Full size image Finally, we investigated heritability of broad community descriptors and found that the number of bacterial species (that is, ‘richness’) in the leaf is affected by host genetic variation ( H 2 ~46%; P =0.021), with host SNPs explaining ~8% ( P =0.023) of the phenotypic variance. Among the most significantly enriched biological processes in the results from GWAS ( Table 2 ) are categories related to trichomes, which modify water use, leaf reflectance and temperature [32] . In the case of plant defense, trichomes tend to discourage insect herbivory [33] , [34] and have been reported to facilitate infection by some species of fungi, both by catching spores [35] and by giving fungi a means to proliferate on the leaf [36] . It is not clear how trichomes shape the bacterial community, but it is interesting to note that bacterial species richness does not change with the number of trichomes on a leaf [10] ( P =0.32, simple linear regression), unless the plants were induced with the defense hormone jasmonic acid ( β =−0.13, R 2 =0.06; P =0.026). It is thus tempting to speculate that richness in the leaf bacterial community is shaped by other plant enemies (for example, insects, fungi) that vector bacteria or trigger defense responses. An additional difficulty is that the pathways responsible for trichome and cuticle synthesis overlap [37] , and mutants in cuticle formation host altered microbial communities [9] . Deciphering how hosts shape bacterial communities is clearly complex, and one must remain aware of both genetic constraints within the host and impacts of other species. In fact, in the results from GWAS of leaf bacterial richness, the most significantly enriched category involves the reproduction of viruses, implying that these loci are pleiotropic or that leaf-associated bacteria and viruses interact, as has been observed during human respiratory [38] and polio [39] infections. Table 2 Biological categories enriched in the 5% tail from GWAS of the log of species richness ( S ) in the bacterial community. Full size table In summary, our results demonstrate that GWAS can help to identify the loci and host processes that structure microbial communities. However, our results also emphasize the need, moving forward, to consider the role of genetic heterogeneity and interactions among microbes in shaping these communities. The role of life-history traits [40] (that is, plant phenology) and the environment should also be taken into account. Studies of the rhizosphere demonstrate a role of soil type and chemistry in addition to host genetics [3] , [4] , [5] . In our study, we controlled for the environment (Methods), but differences in the environment could cause distinct loci or host processes (for example, Tables 1 and 2 ) to shape the leaf microbiome of A. thaliana at different times or places. Similar patterns have been observed for flowering time, a trait for which few candidate genes are identified in both field and greenhouse conditions [41] . Be that as it may, adjusting for environmental factors improves power in mapping studies [42] , [43] , and an understanding of important environmental factors should improve the ability to predict microbial phenotypes. As sequencing costs continue to decrease, the ability to dissect the host–microbial interactions affecting human disease, agriculture and conservation efforts is finally within reach. Field experiment We sowed four replicates of each of 196 accessions of A. thaliana ( Supplementary Table 1 ) in two randomized blocks (two replicates per accession per block) using a mixture (1:1) of Fafard C2 and Metromix 200 soil. The soil was autoclaved to reduce the number of greenhouse bacteria and fungi on plants, before transferring them to the field. Seeds were watered and then stored in a cold dark room (4 °C) to homogenize germination. After 7 days of stratification, all plants were moved to a glass greenhouse and grown in 12 h of light (20 °C) for 19 days (allowing most accessions to germinate and reach the 4-leaf stage). These plants were then transferred to a field site (42.0831°N, 86.351°W; Southwest Michigan Research and Extension Center, Benton Harbor, MI, USA; 22 October, 2008) known to host a naturalized population of A. thaliana . Within blocks, samples were planted 10 cm apart from one another, and the blocks were separated by 2 m. The plants were watered generously on the day of transplanting, but were otherwise left untreated until the end of the experiment. Weather records for the field station can be found at: http://www.enviroweather.msu.edu/weather.php?stn=swm The following spring (27 March, 2009), we used a sterile technique and flash-froze samples in the field using liquid nitrogen, before transferring them to the lab on ice. Samples were stored at −80 °C until further processing. Isolation of host-associated microbial DNA Before DNA extraction, we removed the most loosely associated microbes from each rosette, by washing each sample using an earlier approach [13] , [44] . In brief, we washed each sample first in 0.1 M potassium phosphate buffer, pH 8.0, then in 70% ethanol and finally in sterile water; the water wash was repeated three times. Samples were vortexed (20 s) and centrifuged between each wash before the supernatants were discarded, presumably leaving the most tightly associated members of the epiphytic communities, as well as the endophytic communities. The samples were then extracted using Mo Bio’s Ultra-clean htp-96-well Plant DNA Isolation Kit. To increase cell lysis, we repeated the manufacturer’s recommended freeze-thaw method three times before DNA extraction. DNA was stored at −20 °C until used in PCR. Amplicon library preparation and sequencing (16S and ITS) To characterize the bacterial and fungal communities of A. thaliana , each sample was used as a template to PCR amplify phylogenetically informative regions of 16S (bacteria) and ITS-1 (fungi). We used 454 FLX Titanium emPCR Kits (Lib-L) for all sequencing. Bacteria . To survey bacterial communities, GS FLX Titanium Primer B (5′-CCTATCCCCTGTGTGCCTTGGCAGTCTCAG-3′) was attached to 799F (5′-AACMGGATTAGATACCCKG-3′) [45] ; Primer A (5′-CCATCTCATCCCTGCGTGTCTCCGACTCAG-3′) was combined with a 12-bp error-correcting barcode [46] , a 2-bp linker (5′-AT-3′) and the reverse primer 1193R (5′-ACGTCATCCCCACCTTCC-3′) [13] . Together, 799F and 1193R amplify the hypervariable regions V5, V6 and V7 of the 16S gene. Fungi . To amplify ITS-1, Primer B (above) was attached to the fungus-specific ITS1F (5′-CTTGGTCATTTAGAGGAAGTAA-3′) [47] ; Primer A included a 12-mer barcode, a 2-bp linker (CA) and ITS2 (5′-GCTGCGTTCTTCATCGATGC-3′) [48] . Each sample was PCR-amplified in triplicate, and each 25-μl reaction contained 2-μl genomic DNA, 10-μl 2.5x HotMasterMix (5-Prime) and 0.2 μM of each primer. PCR conditions included an initial denaturing step at 94 °C for 2.5 min, followed by 30 cycles of a denaturing step (94 °C for 30 s), an annealing step (55 °C for 40 s) and an extension step (68 °C for 40 s). A final extension step at 68 °C was performed for 7 min before storing the samples at 4 °C. When necessary, PCR dropouts were re-amplified. All samples were quantified using Picogreen (Invitrogen), and these barcoded libraries were pooled to equimolar concentrations. 799F and 1193R exclude chloroplast DNA [45] . To exclude the remaining mtDNA, we captured the phylogenetic target (~505 bp including the above primers) using a 2% agarose gel. Although this approach is effective in minimizing the amplification of host DNA, it likely misrepresents the abundances of several interesting taxa [45] , such as the Cyanobacteria. The gel slices were extracted (QIAGEN’s QIAquick), and samples were further purified with Ampure magnetic purification beads (Agencourt). Finally, samples were quantified using the Qubit dsDNA HS Assay Kit (Invitrogen) and sequenced using 454 FLX Titanium based-chemistry (Roche Life Sciences). 16S/ITS1 rDNA data processing We denoised all of the SFF files generated from pyrosequencing using AmpliconNoise (version 1.25) [17] and QIIME (1.3) [49] . We required sequence reads to be <500 bp and used Perseus [17] to minimize the number of chimeras. We initially created 560 bacterial amplicon libraries and 570 fungal amplicon libraries with PCR; denoising these resulted in 555 bacterial and 566 fungal samples. We used the default parameters in QIIME to pick OTUs sharing 97% sequence similarity (using the algorithm, ‘cdhit’ (3.1)). Each bacterial OTU was assigned taxonomic status using the RDP (2.2) algorithm, also implemented in QIIME. To determine the taxonomic affinity of fungal OTUs, we used the software package MARTA [50] . Samples with poor sequencing coverage were omitted from all analyses. We required a minimum of 800 reads per bacterial sample and 200 reads per fungal sample; this resulted in 512 bacterial and 549 fungal samples. To correct for differences in sequencing effort (coverage), each sample was resampled to either 800 reads (for bacteria) or 200 reads (for fungi). However, all samples were resampled to contain 200 reads before making comparisons between the bacterial and fungal communities (for example, Supplementary Fig. 4 ). Because the samples were grown in different blocks (above), PCR-amplified in separate 96-well plates and sequenced on separate picotiter (ptp) plates, we took into account these covariates in the analyses described below. Microbial analyses Associations among microbes . To perform Kendall’s Test, we used the kendall.global function in the R -package [51] vegan [52] . Ordination techniques . The function rda (scale=T) in vegan was used to perform PCA, while cca was used for CCA. decorana was used to perform detrended correspondence analysis (DCA). To test the hypothesis that accessions of A. thaliana differ with respect to the composition of their microbial communities, which we characterized with these ordination techniques, we used the functions envfit (for unconstrained ordination techniques) and anova.cca (for ordinations produced by CCA). To investigate whether host genetic differences are easier to discern for well-sequenced taxa than rare taxa (that is, due to species turnover among rare species in the microbial community, sequencing artefacts or some other mechanism), we ordered the species matrix by total (maximum) sequencing coverage per OTU. We prefer to characterize well-sequenced taxa as ‘most heavily sequenced OTUs’ rather than ‘most abundant’ because of common technical artefacts (due to primer biases or RNA operon count differences, and so on). In brief, envfit identifies the direction in multi-dimensional ordination space that is maximally associated with an environmental variable (here, host genotype, or accession_id). The goodness-of-fit statistic is r 2 that is equal to 1−(ss w /ss t ); ss w is the within-group sum of squares and ss t =the total sums of squares. To assess the significance of this association, we permuted the data 999 times and counted the number of times that these simulated r 2 values matched or exceeded the observed r 2 value (including the observed r 2 value, which is assumed to be an observation from the null distribution). To determine whether ordinations produced with CCA are shaped by host-genotype, we used the function anova.cca . This function also relies on permutation tests, but does so to determine how often the observed constrained inertia (the constraint being host-genotype) is exceeded when the data are randomly permuted. Genome-wide association studies We used a mixed-model approach [21] , [22] as implemented in the mixmogam package [23] to account for the complex pattern of relatedness among our accessions for all GWAS. To estimate a genome-wide P value threshold, we performed permutations, where we re-ran association scans (genome-wide) using a linear transformation of the phenotype values. Our method controls for population structure using an approach similar to ref. 53 ; however, instead of simulating phenotypes under the null, we permute the transformed phenotype values. This allows us to also control for false positives that can arise if the residuals do not come from a Gaussian distribution. The transformation matrix is the Cholesky decomposition of the inverse phenotypic covariance matrix, as estimated from the mixed model. By applying this linear transformation to the phenotype values, the resulting vector contains values that are expected to be uncorrelated; we randomly permute these to obtain a new vector that we transform as described in ref. 53 , that is, using the Cholesky decomposition of the phenotypic covariance. As we use efficient mixed models and we only need to transform the phenotypes and the genotypes once, the time complexity of the permutation is O(n 2 m+knm) , where n is the number of individuals, m is the number of genotype variants tested and k is the number of permutations. We performed k =100 permutations for each trait. Phenotypes . To correct for differences in sequencing effort among samples, all data were resampled to either 800 reads (bacterial community) or 200 reads (fungal community) before conducting GWAS using common SNPs (minor allele frequency ≥5%). To identify loci underlying variation in the structure of the bacterial and fungal communities, we considered each (separate) community as an aggregate. The raw data from each community were Hellinger [54] transformed (that is, the OTUs in each sample were expressed as a fraction of the sampling effort and then square-root transformed) before PCA was performed on the most heavily sequenced members of these communities. To be consistent with the results illustrated in Fig. 1 , we analysed the top 2% of the fungal community and the top 50% of the bacterial community. However, we noticed that we could explain a larger fraction of the variance (both from PCA and from SNPs) by analysing smaller fractions of the bacterial community, due to species turnover in the community and the different number of variables considered by PCA. We also conducted GWAS after analysing each microbial community using CCA on the top 2% of the bacterial community and top 3% of the fungal community; DCA was performed on the top 5% of the fungal community and the top 2% of the bacterial community. In general, many researchers prefer CCA over PCA because it is more robust to the so-called ‘horsehoe effect’; its drawback is that eigenvalues from CCA are not as easily interpreted as in PCA. The top five eigenvectors from CCA and PCA were analysed in GWAS. Only four axes (DCA1–4) are output from decorana ( vegan 's function to perform DCA). To evaluate the association between these SNPs and the abundance of individual bacterial or fungal OTUs, each species matrix was either square-root transformed or analysed as the presence/absence of the 100 most heavily sequenced OTUs in each community. As above, we used the vegan function cca to ‘partial-out’ the technical confounders ( cca performs QR decomposition) block, picotiter plate and PCR plate, using the residuals from cca as phenotypes in GWAS, similar to earlier PCA-based approaches [55] . To identify loci associated with bacterial species richness [56] (diversity of order 0), the number of species within each sample was tallied and log-transformed; technical confounders (above) were regressed out before conducting GWAS. Because RNA operon counts differ among species, and bias results from PCR, we avoided estimating ‘true’ diversity (diversity of order 1), which is often calculated using Shannon diversity. The most common results from GWAS . To identify genomic regions shared in the top results from these GWAS, we combined GWAS analyses of the colonization (presence/absence) and proliferation (abundance) for each OTU into one data set. To do so, we combined P values from GWAS using Brown’s method [57] , which is similar to Fisher’s combined P value approach, but suitable for correlated data sets (for example, the P values from these two analyses). We split the results from each analysis into 10-kb windows (yielding 11,614 windows). Then, to make the results comparable across GWAS, we ranked and calculated an empirical P value for each window. Next, we determined the amount of overlap in the top results ( P ≤0.001, empirical P value) from GWAS of individual OTUs in each community. To determine the significance of observed sharing, we used 100,000 simulations to construct a null distribution; each observation in the null was based on selecting 11 ( P ≤0.001) windows from each of 100 simulated GWAS results (that is, 100 OTUs). We then counted the number of times a window was shared ‘x’ or more times. To assess the probability of observing the same genomic region in the bacterial and fungal analyses, we sampled from 200 simulated GWAS results (that is, 100 OTUs from each community). Enrichment of GO-categories in the results from GWAS To determine which biological processes underlie variation in the composition of A. thaliana ’s microbial community, we tested for an overrepresentation of gene ontology (‘goterm’) categories [25] ( ftp://ftp.arabidopsis.org/home/tair/Ontologies/Gene_Ontology/ ) in the top results from GWAS. We omitted gene models with low confidence (evidence code: ‘inferred from electronic annotation’ (IEA)) and any biological category represented by only one gene model, leaving 3,588 unique GO-terms. Next, we split the results from GWAS into 10-kb windows and took the minimum score within that window as the test statistic. We then counted the number of gene models (± 1,000 bp surrounding DNA) within the top 5% of these (windowed) GWAS results. To ensure that we identify ‘broadly’ (that is, genome-wide) enriched categories, we required at least three 10-kb windows to contain gene models from the gene set category. To account for multiple testing, all P values were corrected using Storey’s approach [24] at an FDR level of 10%. To determine the probability of observing a GO-term enriched in the results from GWAS multiple times (as illustrated in Table 1 ), we simulated gene set enrichment analyses. That is, we used 100,000 permutations to construct a null distribution where each observation in the null was constructed by randomly selecting (and tallying), 100 times (that is, 100 OTUs), the same number of GO-terms significantly enriched in the analyses of each OTU. The P values reported in Table 1 reflect the number of times that a biological category is shared x or more times in this null distribution. Accession codes: The 454 pyrosequencing data have been deposited in the European Nucleotide Archive (ENA) Sequence Read Archive with accession code PRJEB7247 . GWAS results are available at the Dryad Digital Repository: http://doi.org/10.5061/dryad.8sm01 . How to cite this article: Horton, M. W. et al. Genome-wide association study of Arabidopsis thaliana leaf microbial community. Nat. Commun. 5:5320 doi: 10.1038/ncomms6320 (2014).